Top-down fabricated silicon nanowires under tensile elastic strain up to 4.5% Strained Si nanowires are among the most promising transistor structures for implementation in very large-scale integration due to of their superior electrostatic control and enhanced transport properties. Realizing even higher strain levels within such nanowires are thus one of the current challenges in microelectronics. Here we achieve 4.5% of elastic strain (7.6 GPa uniaxial tensile stress) in 30 nm wide Si nanowires, which considerably exceeds the limit that can be obtained using SiGe-based virtual substrates. Our approach is based on strain accumulation mechanisms in suspended dumbbell-shaped bridges patterned on strained Si-on-insulator, and is compatible with complementary metal oxide semiconductor fabrication. Potentially, this method can be applied to any tensile prestrained layer, provided the layer can be released from the substrate, enabling the fabrication of a variety of strained semiconductors with unique properties for applications in nanoelectronics, photonics and photovoltaics. This method also opens up opportunities for research on strained materials. One of the great challenges to further improve the scaling down of silicon metal oxide semiconductor field effect transistors (MOSFETs) involves the increase of carrier mobility in the channel while maintaining electrostatic integrity [1] , [2] . The stringent electrostatic requirements have been met in ultra-short transistors by multigate geometry, where the optimum configuration is the nanowire (NW)-like architecture with a wrapped gate [2] , [3] . Mobility enhancement is in turn a very attractive option because it improves device performance beyond the benefits provided by scaling [1] . Mobility enhancement can be achieved by altering the properties of silicon through strain-induced manipulation of the band structure, which modifies the effective masses and phonon scattering within the channel [4] . For these reasons, silicon NWs with strained channels are promising candidates for the next generation of MOSFETs [5] . The main strain-engineering approach currently pursued by the microelectronics industry is based on the deposition of stressor layers on top of transistors. Because the dimensions of current scaled transistors are becoming smaller than the required thickness of such an overlayer, it is difficult to implement this approach into smaller nodes while providing uniaxial tensile stress higher than the presently obtained ~2 GPa (corresponding to ~1.2% strain) [4] , [6] . Indeed, the integration of strain levels higher than those currently available into silicon NWs is recognized as a major milestone for the front end silicon technology at smaller nodes [7] . An alternative way to produce strained silicon is to grow a thin pseudomorphic silicon cap over a strain-relaxed SiGe virtual substrate, which is a graded SiGe thick layer grown on a bulk silicon substrate to control the dislocation density [8] . The defect density and the biaxial tensile strain of the silicon cap depends on the germanium content of the SiGe layer; for example strained silicon with 0.8% strain (20% Ge content) has sufficiently low defect density of about ~10 4 cm −2 . Strained silicon layers grown on higher germanium content buffer layers [9] (Ge >45%) could provide higher strain levels, but the drawback is that the dislocation density would increase to an unacceptable level. Recently, silicon NWs with high uniaxial stress of ~2 GPa (~1.2% strain) have been demonstrated by patterning suspended NWs on highly strained silicon on insulator (SSOI) [10] . These substrates are fabricated by transferring the strained silicon layer from a virtual substrate to an oxidized silicon handle wafer via wafer bonding [11] . The NWs patterned on highly strained silicon layers are released from the buried SiO 2 by wet chemical etching, relaxing the free surfaces while preserving the initial longitudinal strain. Up to two times enhancement in transconductance has been reported for transistors built with such highly strained NWs in respect to those made on conventional silicon substrate [10] . Micro electromechanical system loading has been proposed as an alternative to produce very high longitudinal strain in vapour liquid solid grown ‹111› oriented silicon NWs [12] . In this method, the NW is longitudinally stretched by releasing a prestrained contact cantilever. Although this technique has produced silicon NWs with strain up to ~3.5%, it is still limited for very large-scale integration (VLSI) due to the intrinsic doping of the NW, the use of gold catalysts, the non ideal crystal orientation, the dimensional variability, the large size of the micro electromechanical system and most importantly, the difficulty of controlling the strain. Preconditions for Si microelectronic industry are strict and require compatibility to VLSI substrates, processes using few processing steps and flexibility to a variety of layered systems. In this work, by patterning and releasing dumbbell-shaped bridges from thin biaxial tensile SSOI substrates, we extend the above approaches to fabricate high-quality suspended silicon NWs with longitudinal strain up to ~4.5% (~7.6 GPa uniaxial tensile stress). We use the word 'bridge' to describe an entire structure, including a narrow central NW together with its supporting suspended pads. We utilize a fabrication process that is fully compatible with mainstream complementary metal oxide semiconductor (CMOS) technology. Our bridges are fabricated from SSOI substrates, but the concept can be generalized and used for any tensile strained layer, including free standing defect free Si/SiGe heterostructure membranes [13] . We show that the strain can be controlled accurately by designing the dimensions of the bridge, producing a uniform longitudinal strain in the NW. Further, we demonstrate the extension of the concept to multi-NWs. Strain enhancement in dumbbell-shaped Si nano structures Necked samples are generally used in mechanical tensile tests to control the localisation of the stress and, eventually, the break point [14] . Here dumbbell-shaped structures are used to increase the strain of equibiaxially tensile-stressed SSOI. We reduce the cross-sectional area of the samples, thereby concentrating the tension to the central nanometre sized part of the structure. The starting strain in the equibiaxially tensile-stressed silicon layer amounts to ε 0 ~0.8% as verified by micro Raman measurements. We use SSOI with an intermediate strain because its defect density is lower than that of highly strained SSOI. We patterned dumbbell-shaped structures with different dimensions on 13 nm thick SSOI followed by etching the buried SiO 2 . The bridges were patterned in the ‹110› orientation, which, for strain levels higher than 1%, induces higher electron mobility than biaxial strain [15] . The five dimensions displayed in Fig. 1a classify the resulting suspended bridges: the central NW length A , the overall bridge length B , the NW width a and the pad width b . An additional parameter shown in Fig. 1a is the length L etched underneath the buried oxide, beyond the outer frame of the structure. The released bridges relax in the transverse directions [16] while transferring longitudinally strain from the two pads to the NW located at the bridge centre. Assuming a constant silicon layer thickness, the cross-sectional dependency of the stress distribution used to determine the strain enhancement in the NWs can be reduced to a dependency on the length ratio, ( B − A )/ A , and the width ratio, b / a . 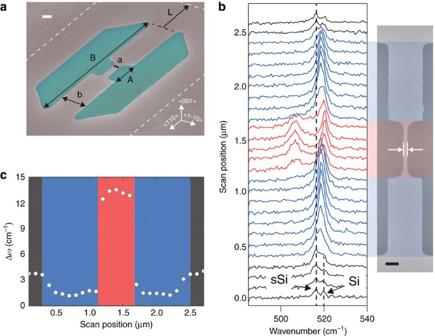Figure 1: Microscopy images of the NWs and Raman spectroscopy mapping. (a) Coloured SEM picture of a suspended strained Si dumbbell bridge with a 200 nm narrow and 13 nm thin NW. The dimensionsA,B,a, andbrefers to the NW length, the bridge length, the NW width and the pad width, respectively. The dimensionLcorresponds to the length of the etching underneath the outer frame, represented by the white dashed line. The scale bar represents 300 nm. (b) Raman line scan measurement of a bridge withA=0.6 μm,B=2.4 μm,a=30 nm andb=360 nm. A SEM picture of the measured bridge is displayed on the right. The Si peak from the substrate is located at 520.0 cm−1, whereas the peaks from the biaxial-strained layer and the uniaxially strained NW are at 514.5 and 506.1 cm−1, respectively. The red and blue shaded areas indicate the NW and pad, respectively. The black scale bar represents 100 nm, whereas the distance between the white arrows indicates that the wire has 30 nm width. (c) Raman shift of the strained Si peak in respect to relaxed Si as a function of the longitudinal position along the bridge. The red and blue shaded areas indicate the position of NW and pad, respectively. The strain enhancement ε x / ε 0, defined as the ratio of strain along the NW ε x divided by the initial strain ε 0 of the layer, is related to the dimensions of the bridge according to (see details in Supplementary Methods ), Figure 1: Microscopy images of the NWs and Raman spectroscopy mapping. ( a ) Coloured SEM picture of a suspended strained Si dumbbell bridge with a 200 nm narrow and 13 nm thin NW. The dimensions A , B , a , and b refers to the NW length, the bridge length, the NW width and the pad width, respectively. The dimension L corresponds to the length of the etching underneath the outer frame, represented by the white dashed line. The scale bar represents 300 nm. ( b ) Raman line scan measurement of a bridge with A =0.6 μm, B =2.4 μm, a =30 nm and b =360 nm. A SEM picture of the measured bridge is displayed on the right. The Si peak from the substrate is located at 520.0 cm −1 , whereas the peaks from the biaxial-strained layer and the uniaxially strained NW are at 514.5 and 506.1 cm −1 , respectively. The red and blue shaded areas indicate the NW and pad, respectively. The black scale bar represents 100 nm, whereas the distance between the white arrows indicates that the wire has 30 nm width. ( c ) Raman shift of the strained Si peak in respect to relaxed Si as a function of the longitudinal position along the bridge. The red and blue shaded areas indicate the position of NW and pad, respectively. Full size image where C is a correction factor to account for the influence of etching underneath the frame. The factor C is discussed later. This expression follows readily from the consideration of a local minimum of the elastic energy, which is achieved by elastic relaxation of the pads (reduction of the free energy) at expense of expansion of the inner NW part, which increases the elastic energy therein. Note that equation (1) is purely a geometrical relation, independent of material properties. Micro Raman experiments and finite element methods Micro Raman measurements along a suspended bridge with a 30 nm-wide NW give clear evidence that the strain in the NW is enhanced by the elastic relaxation of the contact pads ( Fig. 1b ). A typical Raman spectrum of the SSOI layer features two peaks at 520.0 cm −1 (corresponding to bulk cubic silicon), and at 514.5 cm −1 (corresponding to the 0.8% biaxially tensile-strained Si layer). In the contact pad of the suspended bridge, the strained silicon peak shifts towards that of the cubic silicon as an indication of strain relaxation, whereas in the NW the peak shifts towards lower wavenumbers indicating a strain increase. The Raman peak shift Δω was determined by deconvolution of the strained and unstrained cubic silicon signals extracted from the line scan measurements ( Fig. 1c ). Within the resolution of our Raman instrument, the values of strain are constant along the NW yielding a value of about 13.9 cm −1 . The strain ε x along ‹110› direction is calculated from the Raman shift Δω through the following semi-empirical equation for uniaxially stressed Si [17] : where S 11 , S 12 , and S 44 are the silicon compliance tensor entries [17] . From equation (2) the longitudinal strain in the 30 nm-wide NW displayed in Fig. 1b is about 4.0%. A detailed analysis of the strain components in the silicon bridges is found by finite element simulations ( Fig. 2a,b ), which confirms that the longitudinal tensile strain ε x is homogeneously distributed in the NW and amounts ~4.0%, whereas it partially relaxes to about 0.4% in the contact pads. The transverse strain components ε y and ε z of the NW are negative ( Fig. 2b ) as expected. 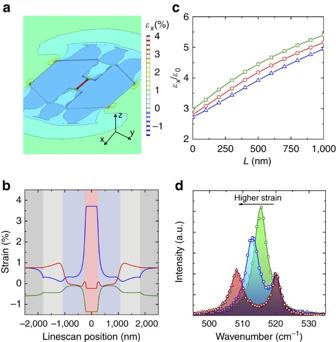Figure 2: Finite element strain simulations and Raman measurements. (a) 3D finite element simulation of the longitudinal strain componentεxof a bridge with dimensions as shown inFig. 1b;A=0.6 μm,B=2.4 μm,a=30 nm,b=360 nm andL=600 nm, whereA,B,aandbrefers to the NW length, the bridge length, the NW width and the pad width, respectively, andLto the under-etched length. (b) Simulated strain components alongx=‹110› (blue),y=‹1–10› (green) andz=‹001› (red) as a function of the line scan position along the length of the bridge displayed in (a). The shaded areas represent the NW (red), pads (blue), under-etched region (light grey) and biaxially stressed layer (dark grey). (c) Strain enhancement in the NW as a function of the under-etching lengthL, for a bridge withb/a=5,B/A=4 andB=2,400 nm. The simulation was performed for wires with 50 (green square), 100 (red circle) and 200 (blue triangle) nm widths. (d) Raman spectra of Si NWs with widthsa=125 (green square), 375 (blue circle) and 725 (red triangle) nm from bridges withA=0.6 μm,B=2.4 μm andb=1.0 μm. Figure 2: Finite element strain simulations and Raman measurements. ( a ) 3D finite element simulation of the longitudinal strain component ε x of a bridge with dimensions as shown in Fig. 1b ; A =0.6 μm, B =2.4 μm, a =30 nm, b =360 nm and L =600 nm, where A , B , a and b refers to the NW length, the bridge length, the NW width and the pad width, respectively, and L to the under-etched length. ( b ) Simulated strain components along x =‹110› (blue), y =‹1–10› (green) and z =‹001› (red) as a function of the line scan position along the length of the bridge displayed in ( a ). The shaded areas represent the NW (red), pads (blue), under-etched region (light grey) and biaxially stressed layer (dark grey). ( c ) Strain enhancement in the NW as a function of the under-etching length L , for a bridge with b/a =5, B/A =4 and B =2,400 nm. The simulation was performed for wires with 50 (green square), 100 (red circle) and 200 (blue triangle) nm widths. ( d ) Raman spectra of Si NWs with widths a =125 (green square), 375 (blue circle) and 725 (red triangle) nm from bridges with A =0.6 μm, B =2.4 μm and b =1.0 μm. Full size image The impact of the etching underneath the frame on the strain of the NW estimated through finite element simulations is quantified in Fig. 2c , which shows bridges with constant cross-sectional ratio b / a =5 for different b and a values. We observe experimentally and in simulations that extending the under etching length L ( Fig. 1a ) results in a substantial increase of the strain in the wire. The effect is weakly dependent on the widths of the bridge at constant cross-sectional ratio ( Fig. 2c ). An enhancement also occurs for the case where a approaches b , when, strictly speaking, no dumbbell-like structure is formed (see Supplementary Discussion ). Instead, the substrate-released bridge resembles a dumbbell with b >> a , which led us to approximate the correction factor in equation (1) by C =( B +2 L )/ B , where L is experimentally determined by scanning electron microscopy (SEM) inspection ( Supplementary Discussion ). Strain dependence on structural dimension We demonstrate that our approach enables fine tuning of the applied strain in the NWs by varying the dimensions of the bridge components, that is, lengths and widths of both pads and wire. Micro Raman spectra of silicon NWs with widths of a =125, 375 and 725 nm from bridges with fixed dimensions A =0.6 μm, B =2.4 μm and b =1.0 μm are shown in Fig. 2d . The longitudinal strain increases for narrower wires as a consequence of the reduced cross section, that is, increased force per area. The decrease of signal strength observed in the spectra of smaller NWs stems from the reduced overlap between the nanostructure and the laser spot (approximately 400 nm diameter). 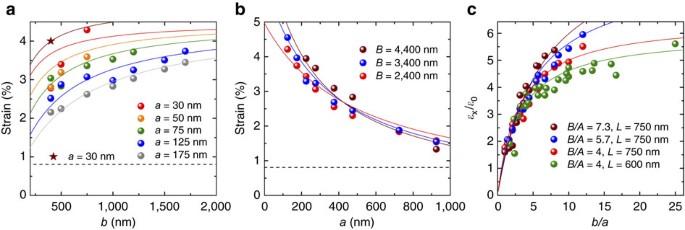Figure 3: Strain dependence on the dimensions of the nanobridges. (a) Longitudinal strain of the NW versus the pad widthbforB=2.4 μm andA=0.6 μm, and different NW widthsa.A,B,aandbrefers to the NW length, the bridge length, the NW width and the pad width, respectively, andLto the under-etched length. The under-etched lengthLis 600 nm for the circle symbol keys, whereas 750 nm for the star symbol key. The strain of the biaxially SSOI is plotted for reference (dashed line). (b) Strain as a function of the NW widthafor a constant pad widthb=1.5 μm andL=750 nm. The wire length isA=0.6 μm, whereas the bridge length was varied fromB=2.4 to 4.4 μm. The strain of the biaxially SSOI is plotted for reference (dashed line). (c) Strain enhancement versus the ratiob/afor NWs with differentbandavalues. The curved lines were obtained from equation. (1), whereas the points represent experimental measurements. Figure 3a shows the strain of NWs as a function of the pad width for wire widths ranging from 30 to 175 nm. The overall length of the bridge is B =2.4 μm and the length of its NW component is A =0.6 μm. The strain increases up to 4.5% by increasing the pad width or decreasing the NW width. In addition, increasing the length L of the etching underneath the outer frame from 600 to 750 nm for a bridge with a =30 nm results in 1.5 times increase in strain. The results obtained from equation (1) using the above dimensions are also plotted. Figure 3: Strain dependence on the dimensions of the nanobridges. ( a ) Longitudinal strain of the NW versus the pad width b for B =2.4 μm and A =0.6 μm, and different NW widths a . A , B , a and b refers to the NW length, the bridge length, the NW width and the pad width, respectively, and L to the under-etched length. The under-etched length L is 600 nm for the circle symbol keys, whereas 750 nm for the star symbol key. The strain of the biaxially SSOI is plotted for reference (dashed line). ( b ) Strain as a function of the NW width a for a constant pad width b =1.5 μm and L =750 nm. The wire length is A =0.6 μm, whereas the bridge length was varied from B =2.4 to 4.4 μm. The strain of the biaxially SSOI is plotted for reference (dashed line). ( c ) Strain enhancement versus the ratio b / a for NWs with different b and a values. The curved lines were obtained from equation. (1), whereas the points represent experimental measurements. Full size image The strain in NWs with larger widths ranging from 125 to 975 nm and fixed pad width of b =1.5 μm is shown in Fig. 3b . The NW length was fixed to A =0.6 μm, whereas the bridge length varied from B =2.4 to 4.4 μm. In this case, the strain decreases by increasing the NW width a . The strain in the NW increases in respect to the biaxial case even as a approaches b. The strain under this condition is found to be ~1.5% uniformly distributed along the entire bridge, which is consistent with equation (1) taking L as ~750 nm. The strain enhancement versus the cross section ratio for bridges with different a and b and with different length ratios is shown in Fig. 3c . The enhancement amounts up to six times beyond the starting strain and is limited only by fracture of the bridges at strain above 4.5%. We found this limit to be independent of the NW width. The experimental data closely match the prediction of equation (1), which indicates that both the width and strain of the fabricated NWs can be controlled by the design of the bridge. Thus, these data provide strong support for the generality of our approach. Strain enhancement in multi-NWs Furthermore, we extend our approach to the fabrication of strained silicon multi-NWs. Multi-NW silicon transistors have been reported as promising building blocks for high-performance logic inverters, fast ring oscillators and demultiplexers [18] , [19] . These devices offer excellent electrostatic control, and higher drive current than those with single wires [20] . The SEM images of such multi-NWs and the respective Raman spectra are shown in Fig. 4 . The strain increases with decreasing the number of wires, such that for single, double and triple wires, the strain is 3.3%, 3.1% and 2.8%, respectively. Linescan measurements show that every individual NW experiences the same strain as its neighbours. The equal distribution of the strain within the array indicates that the strain enhancement does not generate new dislocations. 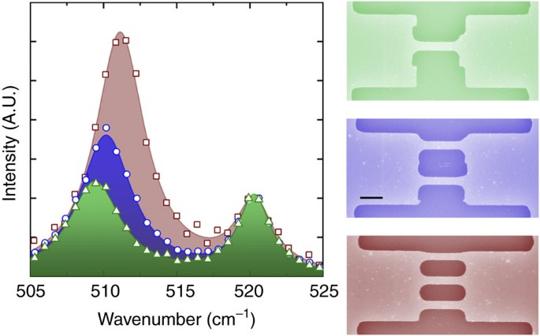Figure 4: Microscopy images and Raman measurements of multi-NWs. False-coloured SEM images (right) of single (green), double (blue) and triple multi-NWs (brown). The scale bar represents 300 nm. Raman spectra of single (green triangle), double (blue circle) and triple multi-NWs (brown square) (left) with strain values of 3.34% (green), 3.09% (blue) and 2.82% (brown), respectively. Figure 4: Microscopy images and Raman measurements of multi-NWs. False-coloured SEM images (right) of single (green), double (blue) and triple multi-NWs (brown). The scale bar represents 300 nm. Raman spectra of single (green triangle), double (blue circle) and triple multi-NWs (brown square) (left) with strain values of 3.34% (green), 3.09% (blue) and 2.82% (brown), respectively. Full size image The mechanical stability and precise positioning control of such highly strained Si NWs in the substrate allows its robust integration into standard transistors. A feasible approach would be, for example, to employ the well-established gate-all-around architeture [10] , [21] . In order to realize this design, we propose employing a gate last process in order to avoid strain relaxation, where activation of source and drain is performed before patterning, and where low temperature conformal deposition of high-κ gate oxide and metal gate is achieved using atomic layer deposition [22] . Although in the present form, the strained NWs are much larger than what is required to VLSI, strain enhancement is solely dependent on the bridge dimensions such that the structures can be scaled down to the limits that lithography methods provide. Yet, our strain technique does not require stressor layers, which may contribute to decrease the contacted gate pitch. Finally, our approach could be used for logic device applications that require low-power MOSFETs but not aggressive scaling such as cellphone circuits. In addition, at 7.6 GPa uniaxial stress, the Si bandgap reduces to about 0.5 eV as verified by 6×6 kp simulations including deformation potentials as provided by the software package Nextnano, which makes our approach very attractive to ultra low power band-to-band tunnelling field effect transistors [23] . From a materials point of view our results are also unique as they demonstrate extremely high uniform strain along x, y and z orthogonal directions (see Fig. 2b ) in contrast to those found in a NW bending geometry [21] . The strain levels are still lower than the theoretical tensile strength of a brittle material, which is expected to be ~ E /10, where E is the Young`s modulus. These levels under uniform tensile stress have only been observed so far by Zhu et al . [24] for epitaxialy grown Si nanowhisker with diameters of about 15 nm, strained using actuators. For the dimensions of our bridges (≥30 nm), we achieved comparable tensile strength, though our NWs were fabricated using a top down approach. This fracture strength (~7.6 GPa) is also equivalent to those obtained in top down fabricated Si NWs from defect free SOI using external actuators [25] . To summarize, we have demonstrated record strains in silicon NWs without actuators or stressor layers but rather by transferring the strain within the suspended structure. It is noteworthy that the achieved strain is higher than those achievable by conventional methods using virtual substrates. Moreover, the method presented here can be applied to any pseudomorphically grown tensile-strained heterostructure material system as it depends purely on geometrical factors. As an example, apart from the application to silicon NWs, this approach could very well be applied to micrometre thick strained Ge layers for photonic applications [26] . Fabrication of the strained Si suspended constricted structures The starting material for the NW fabrication consisted of 13 nm thick equibiaxial tensile-stressed silicon on insulator layer on top of a 145 nm buried oxide layer. Details on the fabrication process and the properties of the SSOI material are described elsewhere [11] . Raman measurements indicated a positive strain of ε =0.8% in the SSOI layer. Electron beam lithography and reactive ion etching using low-energy SF 6 -based plasma were employed to define the dumbbell bridges with different dimensions oriented along the [110] crystal direction. The electron beam lithography resist was removed using Piranha solution. The bridge dimensions were verified by SEM. The buried SiO 2 was etched by directly immersing the samples into buffered hydrofluoric acid (HF) (7:1) during 4–6 min, followed by rinsing in deionized water for 10 min. Raman characterization of strain in the nanostructures Raman spectroscopy was performed using a WITec CRM200 instrument, with a 532 nm excitation and spectral resolution of 0.3 cm −1 . Spectra were collected in backscatter configuration using a X100 magnification optic. All the spectra feature a peak at 520.0 cm −1 , corresponding to the relaxed Si substrate, and a peak found at a position between 505.0 and 520.0 cm −1 , corresponding to strained Si. The relative Raman shift used for the calculation of strain was retrieved by fitting the spectra with two Lorentzians functions and extracting the difference between the peak positions. The s.d. of the peak position is found to be approximately 0.15 cm −1 . How to cite this article: Minamisawa, R.A. et al . Top-down fabricated silicon nanowires under tensile elastic strain up to 4.5%. Nat. Commun. 3:1096 doi: 10.1038/ncomms2102 (2012).